Atomistic mechanism for the activation and desensitization of an AMPA-subtype glutamate receptor Ionotropic glutamate receptors (iGluRs) mediate fast excitatory synaptic transmission in the central nervous system. Upon agonist binding, an iGluR opens to allow the flow of cations and subsequently enters into a desensitized state. It remains unclear how agonist binding to the ligand-binding domain (LBD) is transmitted to the transmembrane domain (TMD) for channel activation and desensitization. Here we report molecular dynamics simulations of an AMPA (α-amino-3-hydroxy-5-methyl-4-isoxazole propionic acid)-subtype iGluR in explicit water and membrane. Channel opening and closing were observed in simulations of the activation and desensitization processes, respectively. The motions of the LBD–TMD linkers along the central axis of the receptor and in the lateral plane contributed cooperatively to channel opening and closing. The detailed mechanism of channel activation and desensitization suggested by the simulations here is consistent with existing data and may serve as a guide for new experiments and for the design of pharmacological agents. Ionotropic glutamate receptors (iGluRs) are tetrameric, non-selective cation channels that mediate fast excitatory synaptic transmission in the central nervous system [1] . They are implicated in numerous central nervous system disorders, and are therefore considered as potential drug targets [2] . Among the four subtypes of iGluRs, α-amino-3-hydroxy-5-methyl-4-isoxazole propionic acid (AMPA) receptors are characterized by rapid activation and deactivation kinetics. The molecular architecture of AMPA receptors is modular and conserved ( Fig. 1 ). An extracellular amino-terminal domain contributes to receptor assembly and surface expression; an extracellular ligand-binding domain (LBD) has a dimer-of-dimers quaternary arrangement [3] , with each subunit consisting of two lobes, D1 and D2, that form a clamshell structure; a transmembrane domain (TMD) contains three membrane-spanning helices (M1, M3 and M4) and a short 'reentrant' helix (M2) per subunit, with the channel pore lined by the M3 helices [4] ; and an intracellular carboxyl-terminal domain contains a variety of sites for post-translational modification and is involved in cytoskeletal interactions. The linking peptides between the LBD and TMD are critical for the coupling of these two domains [5] . 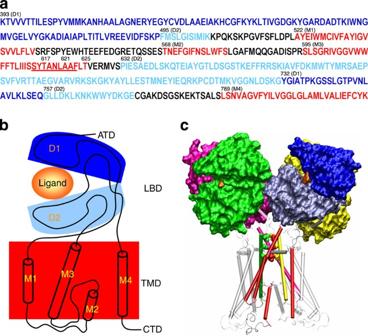Figure 1: Sequence and domain organization of the GluA2 receptor. (a) The sequence is displayed with the D1 and D2 lobes and the transmembrane domain (TMD) in dark blue, light blue and red, respectively. Residue numbers at the starting positions of different regions of D1 and D2 and the TMD helices, and the three pore-blocking positions are given. The highly conserved SYTANLAAF motif at the M3 C-terminal is underlined. (b) The domain organization of a single subunit. The colour code is same as that ina. (c) The tetrameric structure of the receptor in the resting state. The ligand-binding domain (LBD) is shown as surface. The bound ligand in each LBD monomer is shown in orange. The three residues blocking the channel pore (T617, A621 and T625) are shown as space-filling model. TMD helices are shown as cylinders. The front right subunit is shown in the same colour code as ina. For the other three subunits, the D1 and D2 lobes and the M3 helices are in green, magenta and yellow, respectively, but the other TMD helices are in grey. ATD, amino-terminal domain; CTD, carboxyl-terminal domain. Figure 1: Sequence and domain organization of the GluA2 receptor. ( a ) The sequence is displayed with the D1 and D2 lobes and the transmembrane domain (TMD) in dark blue, light blue and red, respectively. Residue numbers at the starting positions of different regions of D1 and D2 and the TMD helices, and the three pore-blocking positions are given. The highly conserved SYTANLAAF motif at the M3 C-terminal is underlined. ( b ) The domain organization of a single subunit. The colour code is same as that in a . ( c ) The tetrameric structure of the receptor in the resting state. The ligand-binding domain (LBD) is shown as surface. The bound ligand in each LBD monomer is shown in orange. The three residues blocking the channel pore (T617, A621 and T625) are shown as space-filling model. TMD helices are shown as cylinders. The front right subunit is shown in the same colour code as in a . For the other three subunits, the D1 and D2 lobes and the M3 helices are in green, magenta and yellow, respectively, but the other TMD helices are in grey. ATD, amino-terminal domain; CTD, carboxyl-terminal domain. Full size image Electrophysiological and crystallographic studies have significantly advanced the structural and functional characterization of AMPA receptors [1] . Much of the focus is on the LBD. The binding of glutamate induces a 25° closure of the clamshell, leading to channel activation [6] . The structures of the isolated LBD in complex with a wide range of agonists, partial agonists and antagonists suggest a correlation between the extent of LBD closure and the degree of channel activation [6] , [7] , [8] , [9] , [10] , [11] . Interlobe twist may also influence agonist efficacy [12] , [13] , [14] . After channel activation, sustained presence of glutamate leads to rapid desensitization [15] , [16] . Desensitization involves significant rearrangement of the LBD; in each dimer the D1 lobes disengage from each other, whereas the D2 lobes are brought closer [17] , [18] . Destabilization of the D1–D1 dimeric interface by mutations disrupting the E486/K493 salt bridge [15] or by G725C and S729C mutations resulting in a disulphide bond in the D2–D2 dimeric interface [17] increases the rate of desensitization; conversely, stabilization of the D1–D1 interface by the binding of allosteric modulators [19] or introducing cation-π interactions [20] slows desensitization. The recent structural determination of the nearly full-length (missing the C-terminal domain) Glu2A AMPA receptor in the resting state was a milestone [21] . For the first time, it became possible to infer the quaternary-level rearrangements of the LBD upon channel activation and desensitization. It was clear that the motions would be much more substantial for the two distal D2 lobes than for the two proximal D2 lobes. Some experimental data exist regarding the gating motions of the LBD–TMD linking peptides [5] , [22] , [23] and the TMD itself [4] . Within the M3-D2 linkers, charge reversal of the conserved residue R628, by an R→E mutation, suppressed desensitization, whereas an opposite charge reversal E→R mutation at the neighbouring position 627 enhanced desensitization [5] . Accessibility of substituted cysteines in the pore-lining M3 helix in the presence and absence of glutamate [4] provides valuable data for testing gating models. However, how the motions of the LBD are transmitted to the TMD and the motions of the TMD itself upon channel activation and desensitization are still largely unknown. In particular, although the structure of the M1–M3 helices of the GluA2 receptor in the resting state superimposes well with the closed conformation of a potassium channel, whether the similarity extends to gating motions of the transmembrane helices is still contentious [4] , [21] . Here we report an atomistic mechanism for the activation and desensitization of the GluA2 receptor suggested by targeted molecular dynamics simulations. Previous simulation studies were limited to isolated regions such as the LBD [13] , [24] , [25] , [26] or LBD–TMD linking peptides [27] . We studied a functioning receptor, consisting of the LBD, the linking peptides and the TMD, in a membrane. We found that, in response to a change of the LBD from the antagonist-bound conformation to the agonist-bound conformation, the motions of the M3-D2 linkers had three components: upward movement as a whole; opposite rotations of the two diagonal pairs; and disparate outward expansions of the two pairs. The upward and outward motions of the linkers lifted the C-terminals of the M3 helices into the water–membrane interface and the disparate lateral motions of the linkers broke the fourfold symmetry of the M3 helices, with one diagonal pair experiencing much greater outward expansion than the other, leading to channel opening. Starting from this putative activated state, the ensuing motions of the LBD–TMD linkers and the TMD upon a change of the LBD from the activated conformation to a desensitized conformation largely reversed those observed upon channel activation. This detailed mechanism of channel activation and desensitization is supported by existing data [4] , [5] , [10] , [22] , [28] , [29] , [30] , [31] . The GluA2 receptor The GluA2 receptor in the present study contained residues K393 to K817, which make up the LBD, the LBD–TMD linkers and the TMD ( Fig. 1 ). Its structure in the resting state (that is, with an antagonist bound to the LBD) was taken from Protein Data Bank (PDB) entry 3KG2 (ref. 21 ). The LBD in this structure has twofold symmetry (consistent with the dimer-of-dimers arrangement), whereas the TMD has fourfold symmetry. Following the nomenclature in the PDB entry, we refer to the two diagonal subunits that have proximal D2 lobes as chains A and C and the other two diagonal subunits, with distal D2 lobes, as chains B and D. In the LBD, chains A and D form one dimer and chains B and C form another dimer. Quaternary arrangements of the LBD tetramers Our overall strategy was to move the LBD from the antagonist-bound conformation first to the agonist-bound conformation and then to the desensitized conformation and observe how the LBD–TMD linkers and the TMD moved in response in the molecular dynamics simulations. The LBD targets in the activated and desensitized states were based on the structures of the isolated LBD bound with glutamate in the absence (PDB entry 1FTJ) [6] and presence of the S729C mutation (PDB entry 2I3W) [17] , respectively. We needed the LBD targets as tetramers, but the isolated LBD structures only unambiguously defined dimers. In building the tetrameric LBD target in the activated state, we preserved its quaternary arrangement in 3KG2 as much as possible. This conservative approach seems justified, as we were able to find a tetramer in the 1FTJ crystal that has a C α root-mean-square deviation (RMSD) of just 4.3 Å from the 3KG2 LBD tetramer. This 1FTJ LBD tetramer served as our target in the activated state. On the other hand, in the 2I3W crystal, the tetramer closest to the putative activated-state LBD has a C α RMSD of 8.4 Å. Again taking a conservative approach, we obtained an LBD tetramer in the desensitized state by superimposing residues P632-E772 (known as S2) of the 2I3W dimer to the corresponding portions of the 3KG2 tetramer twice, once to each of the two dimers of the latter. This putative desensitized LBD has a C α RMSD of 4.4 Å from the putative activated LBD. Sobolevsky et al . [21] also built models for LBD tetramers in the activated and desensitized states by superimposing to the LBD in the resting state, but the superposition was on a monomer basis. We prefer the models obtained on the tetramer (for the activated state) and the dimer (for the desensitized state) bases, as they incorporated information at the quaternary level as much as possible. Still, the movements of P632, the first residue entering D2 after the M3-D2 linker, presented by our LBD models upon activation and desensitization ( Supplementary Fig. S1 ) are qualitatively similar to those presented by the LBD models described by Sobolevsky et al . Gating motions that led to channel activation Starting from the resting state of the GluA2 receptor, we forced the LBD to move from the antagonist-bound conformation to the agonist-bound conformation and followed the resulting motions of the rest of the receptor over a period of 98 ns. In the resting state, the channel pore is blocked at three positions along the M3 helices: T617, A621 and T625 ( Figs 1c and 2a,b ). During the simulation modelling the activation process, these three positions were no longer blocked ( Fig. 2a,b ). We now describe the motions that led to the channel opening. For convenience, we decompose these motions into those along the central axis of the receptor and those in the lateral plane; and we further decompose the lateral motions into expansion or contraction in the radial direction and rotation around the central axis. In describing these motions, we distinguish between the A and C chains (with proximal D2 lobes) from the B and D chains (with distal D2 lobes). 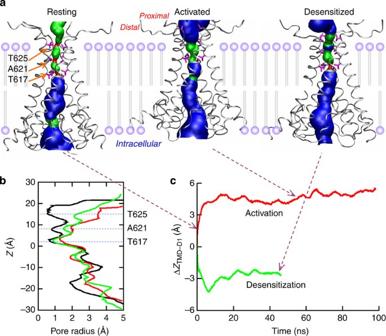Figure 2: Pore-size changes and vertical translation upon channel activation and desensitization. (a) HOLE images45and vertical positions (relative to the membrane) of the transmembrane domain (TMD) in the resting, activated and desensitized states. Residues T617, A621 and T625 are shown as magenta stick. The three states are represented by snapshots at 0.4 and 54.5 ns of the activation simulation and at 45.4 ns of the desensitization simulation. (b) Pore sizes in the resting (black curve), activated (red curve) and desensitized (green curve) states. Here the representative structures of the three states are superimposed on the M3 helices so that pore sizes at the sameZposition along the pore axis can be compared. (c) Vertical translation of the TMD (as represented by T617) relative to the D1 lobes (as represented by K393) of the proximal subunits. Figure 2: Pore-size changes and vertical translation upon channel activation and desensitization. ( a ) HOLE images [45] and vertical positions (relative to the membrane) of the transmembrane domain (TMD) in the resting, activated and desensitized states. Residues T617, A621 and T625 are shown as magenta stick. The three states are represented by snapshots at 0.4 and 54.5 ns of the activation simulation and at 45.4 ns of the desensitization simulation. ( b ) Pore sizes in the resting (black curve), activated (red curve) and desensitized (green curve) states. Here the representative structures of the three states are superimposed on the M3 helices so that pore sizes at the same Z position along the pore axis can be compared. ( c ) Vertical translation of the TMD (as represented by T617) relative to the D1 lobes (as represented by K393) of the proximal subunits. Full size image In the resting state, the connector between the tips (K393 and P632) of the D1 and D2 lobes of a 'distal' LBD monomer is nearly parallel to the central axis (angle at 17°), whereas the counterpart of a 'proximal' LBD monomer is more tilted (angle at 43°; Fig. 3a ). On the other hand, the M3-D2 linker (V626-S631) in a distal subunit is close to being horizontal (and nearly fully extended); in a proximal subunit the M3 helix is longer by one turn compared with the counterpart in a distal subunit, and the remaining short linker (V630-S631) continues in the mostly vertical direction. 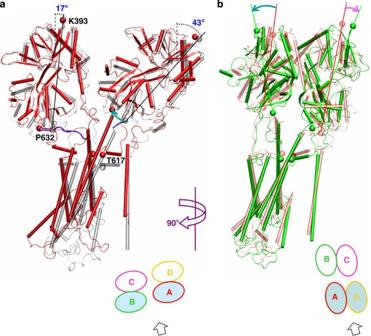Figure 3: Conformational changes of the GluA2 receptor during activation and desensitization shown by two of the subunits. (a) Motions of chains B and A during activation, as shown by a structural comparison between the activated state (in red) and the resting state (in grey) after superimposing on the D1 lobes of the ligand-binding domain (LBD) tetramer. In the resting structure, the tilt angles of the connecters between K393 and P632 in the resting state are shown, and the M3-D2 linkers are highlighted in purple and blue. The directions of rotation of the D2 lobes relative to the respective D1 lobes are shown as magenta and cyan arrows. (b) Motions of chains A and D during desensitization, as shown by a structural comparison between the desensitized state (in green) and the activated state (in light red) after superimposing on the D2 lobes of the LBD tetramer. The directions of rotation of each LBD monomer upon desensitization are shown as cyan and magenta arrows. In bothaandb, the M3 T617 residues are shown as spheres to indicate vertical translation of the transmembrane domain upon activation and desensitization. View directions are indicated by block arrows at the bottom. Figure 3: Conformational changes of the GluA2 receptor during activation and desensitization shown by two of the subunits. ( a ) Motions of chains B and A during activation, as shown by a structural comparison between the activated state (in red) and the resting state (in grey) after superimposing on the D1 lobes of the ligand-binding domain (LBD) tetramer. In the resting structure, the tilt angles of the connecters between K393 and P632 in the resting state are shown, and the M3-D2 linkers are highlighted in purple and blue. The directions of rotation of the D2 lobes relative to the respective D1 lobes are shown as magenta and cyan arrows. ( b ) Motions of chains A and D during desensitization, as shown by a structural comparison between the desensitized state (in green) and the activated state (in light red) after superimposing on the D2 lobes of the LBD tetramer. The directions of rotation of each LBD monomer upon desensitization are shown as cyan and magenta arrows. In both a and b , the M3 T617 residues are shown as spheres to indicate vertical translation of the transmembrane domain upon activation and desensitization. View directions are indicated by block arrows at the bottom. Full size image In our simulation, the closure of the LBD clamshells upon agonist binding led to upward translation of the TMD as a whole, towards the D1 lobes of the LBD ( Figs 2c and 3a ). For the proximal subunits, the closure of the LBD clamshells lifted up the D2 tips and the closely connected M3 helices ( Fig. 3a ). For the distal subunits, the closure of the LBD clamshells lifted up the D2 tips to a lesser extent but moved them significantly away from the central axis (further described below). As a result, the M3 helices had to move up so that the two ends of the M3-D2 linkers were almost even to minimize extending these already nearly fully extended linkers. Therefore, different routes of the proximal and distal subunits led to the same consequence that the M3 helices (and the TMD as a whole) moved upwards by 5 Å towards the D1 lobes ( Fig. 2c ). As a result, the top blocking position, at T625, moved to the water–membrane interface ( Fig. 2a ). Although the decrease in the D1-TMD distance seemed easy to understand given that the D1 and D2 lobes closed up upon agonist binding, it was not immediately clear as to why the TMD had to move upwards to get closer to the D1 lobes. Conceivably, the TMD could have stayed in place but the D1 and D2 lobes moved downwards. The reason that scenario could not occur is that the distal lobes were anchored on top of the membrane (see Fig. 2a ) and so could not move downwards. In the lateral plane, the motions of the M3-D2 linkers (V626-S631) upon agonist binding can be described as outward expansions and opposite rotations of the proximal and distal pairs. 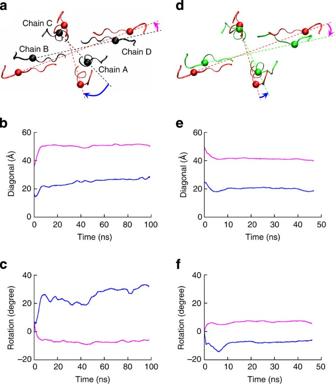Figure 4: Lateral motions of the M3-D2 linkers upon activation and desensitization. (a) Top view of the linkers in the resting (black) and activated (red) states. V630 is chosen as a representative of each linker and is shown as a sphere. The structures of the resting and activated states have been superimposed on the four D1 lobes. (b) Length changes of the AC and BD diagonals upon activation are shown in blue and magenta, respectively. (c) Rotations of the AC and BD diagonals upon activation, shown in blue and magenta, respectively. (d–f) Correspond to (a–c) but are for channel desensitization. Here the structures of the activated and desensitized states have been superimposed on the four D2 lobes, and the linkers in the two states are shown in red and green, respectively. Upon superimposing the four D1 lobes of the activated receptor against the counterparts of the resting receptor, the projected view of the linkers in the lateral plane is shown in Figure 4a . Using residue V630 as a representative, the lengths of the proximal and distal diagonals, plotted in Figure 4b , increased by 9 and 14 Å, respectively. The rotation angles of the proximal and distal diagonals upon activation are plotted in Figure 4c . They reached 30° in the clockwise direction and 7° in the counterclockwise direction, respectively. The opposite rotations brought the angle between the proximal and distal diagonals closer to 90°, which is the value in the fourfold symmetric TMD in the resting state ( Supplementary Fig. S2 ). These lateral motions of the M3-D2 linkers tracked those of P632, the D2 residue directly connected to an M3-D2 linker ( Supplementary Fig. S1 ). Figure 4: Lateral motions of the M3-D2 linkers upon activation and desensitization. ( a ) Top view of the linkers in the resting (black) and activated (red) states. V630 is chosen as a representative of each linker and is shown as a sphere. The structures of the resting and activated states have been superimposed on the four D1 lobes. ( b ) Length changes of the AC and BD diagonals upon activation are shown in blue and magenta, respectively. ( c ) Rotations of the AC and BD diagonals upon activation, shown in blue and magenta, respectively. ( d – f ) Correspond to ( a – c ) but are for channel desensitization. Here the structures of the activated and desensitized states have been superimposed on the four D2 lobes, and the linkers in the two states are shown in red and green, respectively. Full size image In the resting state, the receptor undergoes an abrupt transition from the twofold symmetry of the M3-D2 linkers to the fourfold symmetry of the TMD, as indicated by the angle, θ , between the proximal and distal diagonals ( Supplementary Fig. S2 ). This abrupt transition in θ is maintained in part by the tightly packed M3 helices. In the activated state, the pore is widened, and therefore the M3 helices would have room to move and it would be difficult to maintain an abrupt transition in θ . This conundrum was solved by the opposite rotations of the proximal and distal M3-D2 linkers, whereby the change in θ from the M3 helices to the M3-D2 linkers became much more gradual in the activated state ( Supplementary Fig. S2 ). It appears that the abrupt transition in θ in the resting state builds up a strain, which serves as a driving force for the gating motions of the top portion of the M3 bundle during the activation process. Although the opposite rotations of the proximal and distal M3-D2 linkers allowed the top portion of the M3 bundle to maintain θ close to 90°, the M3 bundle in the activated state still deviated from the fourfold symmetry. The disparate outward expansions of the proximal and distal linkers were mirrored by the lateral motions of the M3 C-terminals ( Supplementary Fig. S3 ). For example, the two proximal T625 residues moved 4.5 Å apart, but the two distal T625 residues moved 9.5 Å apart. In addition, the tilt angles of the proximal and distal M3 helices changed in opposite directions, decreasing in the proximal pair and increasing in the distal pair ( Fig. 5a ). The opposite rotations of the M3-D2 linkers were directly responsible for the opposite changes in the M3 tilt angles. Because the N-terminal portion of each M3 helix is wrapped from the outside by the M1 helix of the same subunit and the M4 helix of an adjacent subunit, the rotation of the M3 helix was largely correlated with the rotations of the latter two helices ( Fig. 5a,b ). 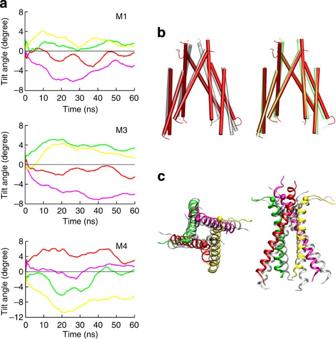Figure 5: Changes in tilt angle and possible bending of three helices upon activation and desensitization. (a) Correlated changes in tilt angle of each M3 helix and the M1 helix of the same chain and the M4 helix of a neighbouring chain during activation. Results for chains A, B, C and D are shown in red, green, magenta and yellow, respectively. (b) Left: comparison of the M3 and M4 helices between the resting state (grey cylinders) and the activated state (red cylinders), after superposition of the M3 helices; right: the same comparison between the activated state (red cylinders) and the desensitized state (green cylinders). (c) Top (left) and side (right) views of the M3 bundle in the resting state (grey spirals) and activated state (red, green, magenta and yellow spirals). Residue T625 is shown as a sphere. Bending of the M3 helix C-terminal in chain B (green spiral) in the activated state is noticeable. Figure 5: Changes in tilt angle and possible bending of three helices upon activation and desensitization. ( a ) Correlated changes in tilt angle of each M3 helix and the M1 helix of the same chain and the M4 helix of a neighbouring chain during activation. Results for chains A, B, C and D are shown in red, green, magenta and yellow, respectively. ( b ) Left: comparison of the M3 and M4 helices between the resting state (grey cylinders) and the activated state (red cylinders), after superposition of the M3 helices; right: the same comparison between the activated state (red cylinders) and the desensitized state (green cylinders). ( c ) Top (left) and side (right) views of the M3 bundle in the resting state (grey spirals) and activated state (red, green, magenta and yellow spirals). Residue T625 is shown as a sphere. Bending of the M3 helix C-terminal in chain B (green spiral) in the activated state is noticeable. Full size image On the basis of the superposition of the M1–M3 helices of the GluA2 receptor with pore-forming helices of a potassium channel, Sobolevsky et al . [21] suggested that, similar to the potassium channel, the GluA2 receptor may open by bending the M3 helices. In our simulation, the C-terminal half of one distal M3 helix showed some sign of bending ( Fig. 5c ), but by no means was the bending solely responsible for the pore opening. As noted previously by Sobolevsky et al. , [4] the C-terminal half of the M3 helix lacks glycines and hence is expected to be relatively rigid. Although in describing the motion of the LBD upon agonist binding we only noted the most prominent feature, that is, the closure of the clamshells, our LBD target for the activated state actually had a small interlobe twist. The latter received attention in recent studies [12] , [13] , [14] . However, we could not tease out the separate contributions of clamshell closure and interlobe twist in our model for channel activation. Gating motions that led to channel desensitization Upon activation, the D1 lobes of an LBD dimer stay engaged but the D2 lobes move apart in closing the clamshells. Upon desensitization, the D1 lobes disengage, whereas the D2 lobes move closer. Consequently, the arrangement of the D2 lobes in the desensitized state partially returns to that in the resting state. The four D2 lobes in our desensitized LBD model superimposed to those in the resting state to 3.5 Å, whereas to those in the activated state to 4.6 Å. In our simulation of the desensitization process, the LBD–TMD linkers and the TMD moved in directions mostly opposite to those observed during the activation process. The reversal in motional directions can largely be attributed to the partial returning of the desensitized D2 lobes to the conformation of the resting state. Now the TMD as a whole moved downwards by 2.5 Å away from the D1 lobes ( Figs 2c and 3b ), pushing the top blocking position T625 back towards the membrane ( Fig. 2a ). In the lateral plane ( Fig. 4d ), the lengths of the diagonals connecting the proximal and distal M3-D2 linkers decreased by 5.5 and 8.5 Å, respectively ( Fig. 4e ), and they rotated counterclockwise by 8° and clockwise by 7° ( Fig. 4f ). The C-terminals of the M3 helices also showed significant inward contraction ( Supplementary Fig. S3 ), leading to the closing of the channel pore ( Fig. 2a,b ). Validation by cysteine modification and coordination data Sobolevsky et al . [4] measured the activation-induced change in accessibility of modifying agents to substituted cysteines along the M3 helices. Previously, we have used such data to validate an activation model obtained by molecular dynamics simulations [32] . Here we use the data of Sobolevsky et al . to test our structure for the activated GluA2 receptor. The basic idea is to compute the solvent accessible areas of a given residue in the resting state and in the activated state, and compare the change against the cysteine modification data at that position. The cysteine modification data show that, upon channel activation, the M3 C-terminal residues L610, I613, S614, T617, N619, A621 and F623 have increased accessibility, whereas L620 has decreased accessibility. 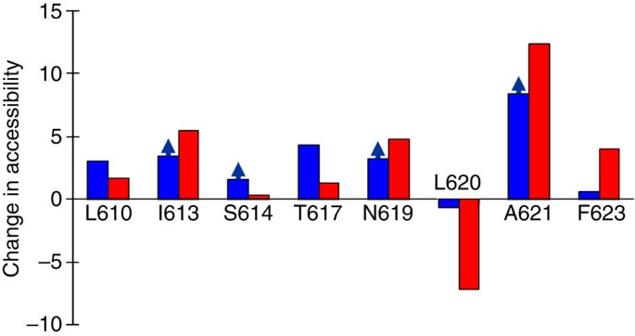Figure 6: Change in solvent accessibility of eight M3 C-terminal residues upon channel activation. The experimental results (blue bars) are ln (kM+/kM−), wherekM+andkM−are modification rate constants of a substituted cysteine by 2-aminoethyl methanethiosulfonate, measured in the presence and absence of glutamate4; arrows for I613, S614, N619 and A621 indicate that the bars present lower bounds. The simulation results (red bars) are differences in solvent accessible area (in Å2) of residues between the activated state and the resting state. The solvent accessible area in the activated state was the average over snapshots between 20 and 54.5 ns of the activation simulation; the counterpart in the resting state was the average over 0–1 ns of the same simulation. As shown in Figure 6 , these changes are reproduced well by the differences in accessible area between our activated structure and the resting structure, with a correlation coefficient of 0.84. L610, I613, S614, T617 and A621 face the pore, so it is easy to see why they became more accessible upon channel activation. N619 and F623 project outwards and are accessible to the solvent on the outside. In our activated model, the outward expansion of M3 pushed these two residues further into the solvent on the outside and hence made them more accessible. On the other hand, L620 also projects outwards but faces the pre-M1 helix in the same subunit ( Supplementary Fig. S4 ). As M3 expanded outwards, the spacing between L620 and the pre-M1 helix was reduced and hence L620 became less accessible. Figure 6: Change in solvent accessibility of eight M3 C-terminal residues upon channel activation. The experimental results (blue bars) are ln ( k M + / k M − ), where k M + and k M − are modification rate constants of a substituted cysteine by 2-aminoethyl methanethiosulfonate, measured in the presence and absence of glutamate [4] ; arrows for I613, S614, N619 and A621 indicate that the bars present lower bounds. The simulation results (red bars) are differences in solvent accessible area (in Å 2 ) of residues between the activated state and the resting state. The solvent accessible area in the activated state was the average over snapshots between 20 and 54.5 ns of the activation simulation; the counterpart in the resting state was the average over 0–1 ns of the same simulation. Full size image Sobolevsky et al . [28] further probed the distances of the four cysteines substituting A621 in the activated state by Cd 2+ coordination. Their data suggest that the four substituted cysteines have twofold symmetry, with two neighbouring pairs close enough for Cd 2+ coordination but the remaining two pairs further apart. Our structure for the activated state agrees very well with this observation (see Supplementary Fig. 3 ): the distances of C β atoms of A621 residues were 4–5 Å between chains A and B and between chains C and D, but 6–7 Å between chains A and D and between chains C and B. On the basis of molecular dynamics simulations, we have obtained atomic-level conformational changes that putatively lead to activation and desensitization of an AMPA receptor. The suggested functional mechanism, involving several unique features, can explain a number of observations on the channel activity of the receptor. 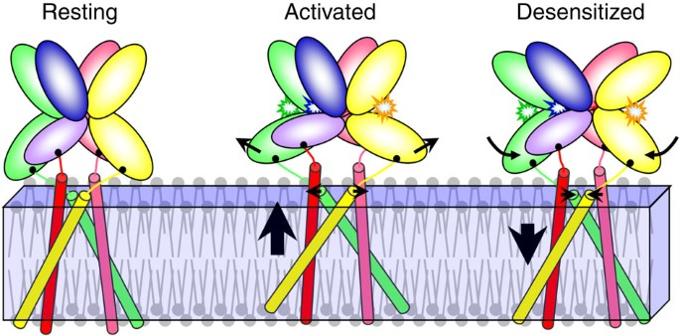Figure 7: Illustration of the proposed mechanism of activation and desensitization. Prominent motions of the ligand-binding domain (LBD) and transmembrane domain (TMD) are indicated by arrows. Upon agonist binding, the distal D2 lobes move outwards, pulling apart the C-terminals of the corresponding M3 helices and lifting up the TMD. In the subsequent desensitization, the LBD monomers rotate inwards, so the arrangement of the D2 lobes partially returns to that in the resting state. Consequently, the C-terminals of the M3 helices move inwards and the TMD translates downwards. The functional mechanism of the AMPA receptor suggested by our simulations is illustrated in Figure 7 . Upon glutamate binding, the closure of the D2 lobes towards the D1 lobes pulls apart the distal pair of M3-D2 linkers and, to a lesser extent, the proximal counterpart. At the same time, the two pairs of diagonal linkers rotate away from each other. As a result, the TMD translates upwards, and the C-terminals of the M3 helices expand outwards, leading to channel opening. Figure 7: Illustration of the proposed mechanism of activation and desensitization. Prominent motions of the ligand-binding domain (LBD) and transmembrane domain (TMD) are indicated by arrows. Upon agonist binding, the distal D2 lobes move outwards, pulling apart the C-terminals of the corresponding M3 helices and lifting up the TMD. In the subsequent desensitization, the LBD monomers rotate inwards, so the arrangement of the D2 lobes partially returns to that in the resting state. Consequently, the C-terminals of the M3 helices move inwards and the TMD translates downwards. Full size image Under sustained presence of glutamate, the two D1 lobes in each LBD dimer disengage and the D2 lobes approach each other, partially restoring the relative arrangement of the latter in the resting state. Consequently, the conformational changes of the LBD–TMD linkers and the TMD in the activation process are largely reversed, leading to channel desensitization. Figure 6 shows that our model for the activated state reproduces well the observed changes in accessibility of key residues upon channel activation. Our mechanistic model also explains other observations on channel activity. Yelshansky et al . [5] investigated the role of the M3-D2 linkers in channel activity and found that reversing the charge on the conserved residue R628 disrupted desensitization, and charge reversal in the opposite direction on the neighbouring E627 enhanced desensitization. They hypothesized that unspecified electrostatic interactions of R628 with the LBD promoted the channel's entrance to the desensitized state, whereas opposite interactions of E627 hindered it. In our structures for the activated and desensitized states, we did not find any systematic differences in short-range or long-range interactions of R628 and E627 with the rest of the receptor. On the other hand, on going from the activated state to the desensitized state, the proximal M3-D2 linkers moved towards the membrane ( Fig. 8a ). Although our simulations were done in a membrane consisting of purely zwitterionic lipids, it can be deduced that, in a cell membrane containing negatively charged lipids, electrostatic interactions of R628 and E627 with nearby phosphate groups of the lipids would be significantly strengthened on going to the desensitized state ( Fig. 8b ). Therefore, a charge reversal of R628 would disfavour the desensitized state, whereas a charge reversal of E627 would have the opposite effect. We thus propose that the electrostatic interactions of R628 and E627 with the membrane explain the mutational effects observed by Yelshansky et al . on channel desensitization. 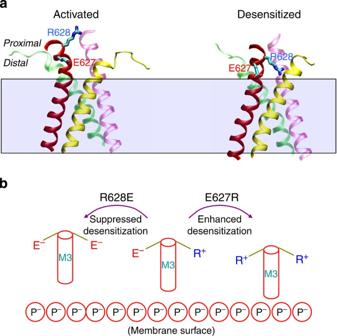Figure 8: Possible involvement of electrostatic interactions with a cell membrane in channel desensitization. (a) Decrease in separation of E627 and R628 residues in a proximal M3-D2 linker from the membrane on going from the activated state to the desensitized state. (b) Cartoon illustrating how electrostatic interactions of charged residues in the proximal M3-D2 linker with the membrane may affect desensitization kinetics. R628E introduces repulsion from the negatively charged membrane, hindering the downward translation of M3 and desensitization, whereas E627R has the opposite effect. Figure 8: Possible involvement of electrostatic interactions with a cell membrane in channel desensitization. ( a ) Decrease in separation of E627 and R628 residues in a proximal M3-D2 linker from the membrane on going from the activated state to the desensitized state. ( b ) Cartoon illustrating how electrostatic interactions of charged residues in the proximal M3-D2 linker with the membrane may affect desensitization kinetics. R628E introduces repulsion from the negatively charged membrane, hindering the downward translation of M3 and desensitization, whereas E627R has the opposite effect. Full size image Using mutagenesis, Balannik et al . [22] identified four residues affecting the binding of two non-competitive antagonists, and showed that these antagonists have lower affinity for the activated receptor than for the resting or desensitized receptor. In the resting GluA2 receptor, the identified residues are clustered around a binding pocket, putatively the binding site of the non-competitive antagonists ( Supplementary Fig. 5 ). In our structure for the activated state, these residues move apart and the binding pocket becomes partially occluded by a portion of the outwardly moved D2-M4 linker, thus explaining the lower binding affinity of the non-competitive antagonists. The extent of LBD closure induced by ligand binding appears to be correlated with the degree of channel activation [1] , [6] , [10] , [21] . Agonists induce the greatest LBD closure and open the channel to the greatest extent; partial agonists induce moderate closure of the LBD clamshells and open the channel to a moderate extent; antagonists keep the LBD in the open conformation and the channel closed. The D2 lobes are connected to the pore-forming M3 helices by the M3-D2 linkers; in our model for channel activation, the closure of the D2 lobes is directly translated into the outward expansion of the M3 C-terminals and channel opening. Therefore, the correlation between the extent of LBD closure and the degree of channel activation is easily explained. A related observation is that single-channel currents show step-like transitions between adjacent conductance levels [10] , [29] , [30] , [31] , suggesting that agonist binding to a subset of the four monomers of the LBD can trigger sub-conductance currents. In our model, closure of a single LBD monomer can lead to outward expansion of the M3 helix in the same subunit, possibly explaining the sub-conductance currents. The four subunits, however, are not equal: the subunits with the distal M3-D2 linkers contribute more to channel conductance compared with the proximal counterparts. The gating motions of the M3 and M4 helices in our model are tightly coupled ( Fig. 5b ). This tight coupling perhaps in part explains why removal of the M4 helix results in loss of channel function [33] . It may also explain the observation that disruption of the interactions between M3 and M4 helices alters channel activation and desensitization kinetics [34] . Several features in the proposed model for the activation and desensitization of the GluA2 receptor are worth noting. First, the distal M3-D2 linkers and M3 helices and their proximal counterparts undergo disparate motions. The distal subunits experience greater outward expansion and inward contraction, and hence contribute more to channel activation and desensitization. Second, our mechanistic model involves the membrane. The distal M3-D2 linkers are anchored on top of the membrane and move outwards within a lateral plane during activation, pulling the M3 helices upwards; the motions are reversed during desensitization. We further propose that long-range electrostatic interactions between charged residues in the M3-D2 linkers and the membrane have a role in channel activation and desensitization. Third, in our model, the motions that directly lead to pore opening and closing are essentially confined to the C-terminals of the M3 helices. It is interesting that the sequence of this region, SYTANLAAF, is highly conserved, raising the prospect that a common gating mechanism may operate for all iGluRs. This prospect is reinforced by the finding that the GluN1-GluN2A heteromeric NMDA receptor has glutamate-binding sites on the GluN2A subunits that are very similar to those in the GluA2 receptor [35] . The GluN2A subunits occupy the distal positions in the M3-D2 linker region, and would thus have a predominant gating role according to our model. Importantly, the Lurcher mutation occurs in the conserved SYTANLAAF motif. The atomistic model developed here for the activation and desensitization of the GluA2 receptor can be further validated by new experiments. For example, the predicted changes in solvent accessibility of residues outside the C-terminal of the M3 helix in our activated and desensitized structures can be tested against accessibility of substituted cysteines. On the basis of the activated and desensitized structures, we can predict how mutations may affect channel activation and desensitization, and the predictions can be interrogated by electrophysiological data. The D1–D1 dimeric interface has been the primary binding site for allosteric modulators [19] . Our activated and desensitized structures open new target sites for designing allosteric modulators. Ligands that show preferential binding to regions of the receptor, such as the LBD–TMD linkers [22] or the TMD, in either the activated state or the desensitized state will allow channel activation and desensitization kinetics to be altered in desired directions. System setup The starting structure of the GluA2 receptor was taken from PDB 3KG2 (ref. 21 ), with all missing side chains and loops built and hydrogen atoms added. The LBD targets in the activated and desensitized states were based on the structures of the isolated LBD bound with glutamate in the absence (PDB entry 1FTJ) [6] and presence of the S729C mutation (PDB entry 2I3W) [17] , respectively. In these isolated LBD structures, K506 and P632 are connected by a two-residue linker (with sequence GT). Comparison with the LBD of the full-length 3KG2 shows that the two-residue linker does not introduce significant distortion. The D2 lobe of 1FTJ and the counterpart of 3KG2 have an RMSD of only 0.8 Å. 3KG2 has a relatively low resolution (3.6 Å), and the resolution of the M3-D2 linkers, which turned out to have a prominent role in our mechanistic model, are probably even lower. However, what matters most to our model is the twofold symmetry of these linkers, which should not be affected by the low resolution of 3KG2. The S729C mutant is regarded as a model for the desensitized state, through destabilizing the D1–D1 dimeric interface, although it may differ subtly from the native structure of the desensitized state [17] . Molecular dynamics simulations Both regular [32] , [36] , [37] and targeted molecular dynamics simulations [38] have been very useful in suggesting gating motions of another family of ligand-gated ion channels, the nicotinic acetylcholine receptors. Targeted molecular dynamics simulations [39] , by making use of mechanistic knowledge, are able to bridge the gap in timescales between regular molecular dynamics simulations (tens of ns) and channel gating (ms). Given the rich information on the conformational changes of AMPA-subtype LBDs, this approach was particularly suited here. In the molecular dynamics simulations, the TMD of the receptor was embedded in a bilayer of 1-palmytoil-2-oleoyl- sn -glycero-3-phosphatidylcholine (POPC) lipids (313 per leaflet) and the receptor–lipid system was solvated by 105,231 water molecules, 114 sodium ions and 118 chloride ions. The extra four anions served to neutralize the whole system, which had a total of 426,461 atoms. The bilayer was prepared by trimming a 2×2 replication of a pre-equilibrated POPC bilayer with 128 lipids per leaflet, downloaded from CHARMM-GUI [40] . NAMD version 2.7b3 (ref. 41 ) was used to run the simulations. Before the simulation of the activation process, the system was energy minimized (1,000 steps), gradually heated to 300 K (over 100 ps under constant NVT ) and equilibrated under constant NPγT (pressure at 1 atm and surface tension at 20 dyn cm −1 (ref. 42 )) for 10 ns. During this process, the backbone atoms of the receptor were restrained (force constant at 20 kcal mol −1 Å −2 ). In the simulation of the activation process, the LBD was steered towards the activated target by an RMSD-based restraint potential (force constant at 20,000 kcal mol −1 Å −2 ). The simulation was run for 98 ns under constant NγPT . The snapshot at 50.9 ns was used to start the simulation of the desensitized process, in which the LBD now was steered towards the desensitized target. This simulation was run for 47.6 ns. Four additional simulations with weaker restraints to the activated and desensitized targets were also run, and the results were similar. Charmm22 all-hydrogen parameters were used [43] , [44] . Periodic boundary conditions were applied, with the particle mesh Ewald method used for treating long-range electrostatic interactions. Constant temperature was achieved by running Langevin dynamics, and constant pressure and surface tension were achieved by the Nose-Hoover Langevin piston method. The SHAKE algorithm was applied to constrain all bonds involving hydrogen atoms, which allowed for an integration time step of 2 fs. How to cite this article: Dong, H. et al . Atomistic mechanism for the activation and desensitization of an AMPA-subtype glutamate receptor. Nat. Commun. 2:354 doi: 10.1038/ncomms1362 (2011).